Real-time QEXAFS spectroscopy measures rapid precipitate formation at the mineral–water interface Reactions at the mineral–water interface are central to numerous geochemical processes and have consequences at local, regional and global scales. They are also important in materials science research. Kinetics greatly influences mineral–water interface reactions; however, there are few kinetic data in real-time and at the molecular scale. Here we report real-time data illustrating the rapid formation of nickel aluminium-layered double hydroxide precipitates at the mineral–water interface in a flow environment in as little as 31–40 min. Layered double hydroxides have a variety of applications in environmental remediation and materials science. The real-time data shown here enhance our fundamental understanding of the kinetics of mineral–water interface processes, such as adsorption, dissolution and precipitation, by illustrating their rapid and simultaneous occurrence in a dynamic environment. Both precipitation and adsorption can occur on the same rapid timescale. The kinetics, mechanisms and thermodynamics of sorption reactions and surface atomic structure control mineral–water interface reactions. Examples include weathering and soil formation, formation of clays and iron oxides, nutrient and trace metal fate and bioavailability, carbon sequestration, acid mine drainage, soil permeability, redox reactions and precipitation processes for environmental remediation [1] , [2] , [3] , [4] , [5] , [6] , [7] , [8] . A molecular-scale understanding of the kinetics and reactions of metal adsorption at the mineral surface is critical not only to geochemical processes but also to colloid chemistry, corrosion science, materials science and in the preparation/manufacture of heterogeneous catalysts [9] , [10] , [11] , [12] . Newly formed surface precipitates, such as hydrotalcite-type layered double-metal hydroxides (LDHs), which form at the mineral–water interface, have versatile roles in important environmental reactions. Layered single or double metal hydroxides are composed of brucite-type hydroxide sheets (octahedral layers) containing one or two metals, respectively. In nickel–aluminium (Ni–Al) LDHs some Ni 2+ is replaced by Al 3+ in the octahedral layers, which gives a positive charge to the layers. The positive charge is balanced by anions. Anions and water molecules are located in between the layers [2] , [11] , [13] , [14] . They can immobilize trace metals in soils, decrease metal bioavailability, control the concentrations of metal contaminants in natural waters and improve design calculations for the geologic storage of contaminated waste; in addition, they are thermodynamically more stable than single-metal hydroxides [2] , [11] , [15] , [16] , [17] . LDHs have a variety of applications including adsorbents, anion scavengers, anion exchangers, polymer stabilizers and nanoreactors [14] . More recently, LDHs have been shown to be important compounds in water oxidation catalysis [18] . Al-based LDHs occurring in soil environments have been identified for reactions with iron(II), cobalt, Ni and zinc [11] , [13] , [19] , [20] , [21] , [22] , [23] , [24] , [25] . Several researchers have used quick scanning X-ray absorption spectroscopy (Q-XAS) batch techniques to investigate redox reactions or iron oxide transformations [26] , [27] , [28] , [29] , [30] at the mineral–water interface, but there are no examples of Q-XAS to illustrate real-time adsorption/precipitation under dynamic/flow conditions. We combine a custom-built flow cell and Q-XAS [31] to study these sorption processes at the clay mineral–water interface in real-time, in situ and at the molecular scale. The flow system in conjunction with Q-XAS reduces artefacts that can occur in batch systems such as re-sorption of products [17] and allows for XAS data collection from the beginning of the sorption reaction. These experiments show the rapid formation of Ni–Al LDH precipitates at the mineral–water interface and highlight the dynamic role the mineral plays during precipitation even on short timescales similar to adsorption. QEXAFS χ (k) and Fourier transformation Data from five experimental runs under varying conditions are described. 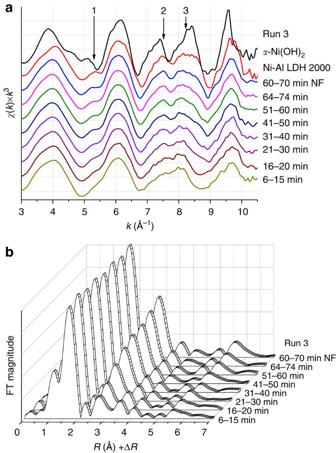Figure 1: QEXAFS data and FT from sample Run 3. (a) Run 3 time series with a comparison of two isostructural compounds, α-Ni(OH)2and Ni–Al LDH13. The characteristic peak reduction caused by the beat pattern at ~8.2 Å−1seen in the LDH is also present in Run 3 at reaction times of 31–40 min and beyond, indicating that an LDH has formed. (b) The radial structure function plot shows increases in the first, second and third metal coordination shell amplitudes throughout the reaction. Figure 1 provides the quick scanning extended X-ray absorption fine structure (QEXAFS) data of Run 3 and the Fourier transform (FT) of those data. It exemplifies the trends common to other runs ( Figs 2 and 3 ). Figure 1 includes a direct comparison with the synthetic isostructural standards α-Ni(OH) 2 and Ni–Al LDH [13] . Several features are indicated by arrows 1, 2 and 3. At ~5.3 Å −1 , arrow 1 indicates a shoulder forming as time progresses. At the beginning of the reaction, the shoulder is not present and then becomes pronounced over time. The shoulder results from focused (linear) multiple scattering paths involving both Ni and Al at a distance of ~6.12 Å −1 in the planar hydroxide layer and is common to many layered single hydroxides, LDHs, and phyllosilicates [11] , [13] , [19] , [32] . 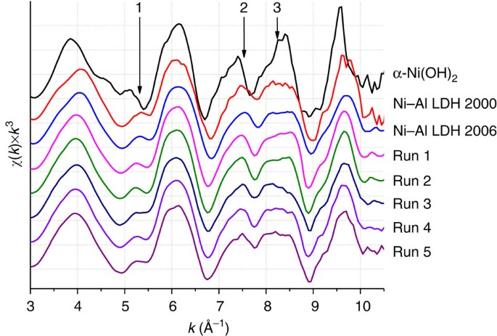Figure 2: A comparison of all samples to standards at the end of each run. Three standards (Ni–Al LDH 2000 (ref.13), α-Ni(OH)2(ref.13) and Ni–Al LDH 2006 (ref.16) illustrate the similarities of the samples to Ni–Al LDH standards. Peak reduction from the beat pattern at ~8.2 Å−1is present in all sample runs and in both LDH standards. α-Ni(OH)2has higher amplitude and peaks at ~8.4 Å−1. Figure 2 compares data at the end of each sample run to three standards. The first two standards are α-Ni(OH) 2 and Ni–Al LDH [13] . The second standard is a different Ni–Al LDH [16] with carbonate interlayer anions. These standards exemplify how all the samples regardless of slight modifications in reaction conditions yield Ni–Al LDH. The peak reduction caused by the beat pattern [13] at ~8.2 Å −1 is present in all sample runs and in both LDH standards. Figure 1: QEXAFS data and FT from sample Run 3. ( a ) Run 3 time series with a comparison of two isostructural compounds, α-Ni(OH) 2 and Ni–Al LDH [13] . The characteristic peak reduction caused by the beat pattern at ~8.2 Å −1 seen in the LDH is also present in Run 3 at reaction times of 31–40 min and beyond, indicating that an LDH has formed. ( b ) The radial structure function plot shows increases in the first, second and third metal coordination shell amplitudes throughout the reaction. Full size image Figure 2: A comparison of all samples to standards at the end of each run. Three standards (Ni–Al LDH 2000 (ref. 13 ), α-Ni(OH) 2 (ref. 13 ) and Ni–Al LDH 2006 (ref. 16 ) illustrate the similarities of the samples to Ni–Al LDH standards. Peak reduction from the beat pattern at ~8.2 Å −1 is present in all sample runs and in both LDH standards. α-Ni(OH) 2 has higher amplitude and peaks at ~8.4 Å −1 . 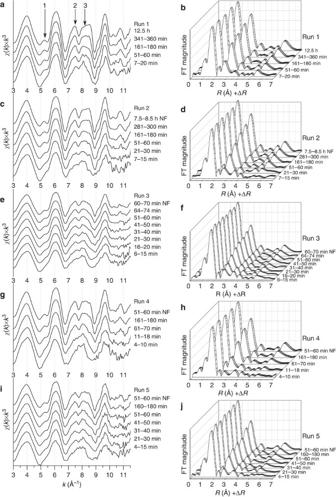Figure 3: QEXAFS and radial structure function plots of all sample runs. Arrows 1, 2 and 3 indicate similar emerging structural changes common to all samples over time despite slightly different reaction conditions. In all EXAFS data, the samples over time develop a peat pattern at ~8.2 Å−1, indicative of Ni–Al LDH13. In all RSF plots, the first Ni–O shell remains at constant amplitude while the first, second and third metal coordination shell amplitudes increase throughout the reaction. Non-flowing conditions are indicated as NF. Runs 1–5 are shown ina–j. Full size image Figure 3: QEXAFS and radial structure function plots of all sample runs. Arrows 1, 2 and 3 indicate similar emerging structural changes common to all samples over time despite slightly different reaction conditions. In all EXAFS data, the samples over time develop a peat pattern at ~8.2 Å −1 , indicative of Ni–Al LDH [13] . In all RSF plots, the first Ni–O shell remains at constant amplitude while the first, second and third metal coordination shell amplitudes increase throughout the reaction. Non-flowing conditions are indicated as NF. Runs 1–5 are shown in a – j . Full size image In all samples, one peak separates into two between 7 and 9 Å −1 . In Fig. 1 , the peak height at ~7.5 Å −1 (arrow 2) becomes equal to that of the peak at ~8.2 Å −1 (arrow 3) starting at 31–40 min and remains so throughout the rest of the reaction. The samples and LDH standards have reduced peaks at ~8.2 Å −1 compared with the α-Ni(OH) 2 standard, which has higher amplitude and peaks at ~8.4 Å −1 . The peak reduction at ~8.2 Å −1 is caused by a beat pattern of destructive overlapping Ni–Ni and Ni–Al photoelectric waves [11] , [33] , [34] and can be used to unequivocally distinguish LDHs from hydroxides [13] . The reduced peak at ~8.2 Å −1 indicates that a Ni–Al LDH has formed by 31–40 min in Run 3. As the reaction progresses, all samples yield similar spectra to the LDH standard at ~8.2 Å −1 during the first 70 min ( Fig. 3 ). Figure 1 also contains the radial structure function of Run 3 uncorrected for phase shift. The amplitude of the first shell at ~1.6 Å remains constant, whereas that of the second shell at ~2.65 Å increases over time. The second shell is dynamic over time in all samples, increasing in amplitude and changing slightly in distance and backscatterer coordination number (CN; Fig. 3 and Table 1 ). The changes in amplitude, distance and CN indicate shifts in the local atomic environment surrounding the central Ni atom. In Fig. 1 , at the beginning of Run 3 (6–15 min), the second shell is small. However, it increases over time as Ni accumulates as Ni–Al LDH that forms in the cell. The sorbent (pyrophyllite) contributes Al [25] . Multiple scattering shells at ~4.9 and ~5.6 Å present in all samples ( Figs 1 and 3 ) are the second and third metal coordination shells in the hydroxide sheet and also increase in height with reaction time. They result from focused multiple scattering in the hydroxide layer and indicate increasing crystallinity over time as they are most prominent at the end of the reaction [13] , [35] , [36] , [37] . Table 1 Structural fitting parameters* for all sample runs and two standards (Ni–Al LDH 3.1 and α -Ni(OH) 2 ) (ref. 13 ). Full size table QEXAFS shell fitting The real-time data include intermediate phases forming before LDH. However, the contribution of several different backscatters around the central Ni atom at various distances complicates analysis of the second shell by the statistical techniques used in EXAFS analysis (for example, reduced chi square ( χ V 2 ) and R-factor). Table 1 gives the structural fitting parameters for all sample runs. The first shell contains oxygen with a CN range of 5.6–6.4. The Ni–O distances ranged between 2.05 and 2.08 Å, with 2.06 Å being the median. The second shell of Ni–Ni ranged from 3.10 to 3.07 Å with the CN ranging from 0.5 to 4. Distances of 3.07–3.08 Å were the median values. Ni–Al LDHs can be identified in the EXAFS data because of the peak reduction at ~8.2 Å −1 caused by the beat pattern [13] . Based on the beat pattern, the time for Ni–Al LDH formation varied from 30 to 70 min of flow ( Fig. 3 ). Analysis of the second shell is complicated by the contribution of several different backscatters around the central Ni atom. In silicated mixed metal hydroxides, for example, a silicated-Ni–Al–LDH, Al substitution for Ni in the octahedral layer and silicon present in a tetrahedral layer simultaneously produce two different backscattered photoelectric waves that are partially destructive and constructive, respectively, with the wave produced by Ni in the octahedral layer. The Ni–Ni and Ni–Al photoelectric waves produced from those atom pairs at ~3.06 Å in the octahedral sheet create partially destructive interference because they are opposite in frequency; however, partially constructive interference occurs between Ni–Ni and Ni–Si when the Si atoms are further away from the absorbing Ni atom and located in a tetrahedral sheet at, for example, 3.21 Å [11] , [13] , [33] , [34] . In addition, impurities (for example, covalently bonded NO 3 − to the hydroxide layer and/or vacancy sites) make it challenging to decide which atoms apart from Ni belong to the second shell using the statistics of χ V 2 , χ 2 and R-factor. Table 1 structural fitting parameters mainly consist of Ni–Ni for second shell fits for those reasons. In addition, using only Ni–Ni for the second shell avoids any false-positive results for Al or silicon scattering paths. For example, χ V 2 values at the end of all sample runs are significantly smaller with the inclusion of silicon and Al into the fit (fitting model B). A decrease in χ V 2 of about two is considered to be significant improvement in the fit [38] . However, when silicon is added to the α-Ni(OH) 2 standard, the χ V 2 value also decreases by more than two times. Perhaps this is owing to similar backscattering frequencies of silicon and the nitrate groups commonly found covalently bonded in single-layered hydroxides [11] , [13] . The α-Ni(OH) 2 standard is known to have no silicon in the interlayer according to the Fourier transform infrared spectra [13] ; however, because silicon can improve the fit there is no confidence to place silicon as a scattering path into unknown samples. Fitting model B yields a statistically better fit without adding additional fitting parameters but is not used at the earlier reaction times because even though the χ V 2 values decrease they do not do so by a factor of two or more. For fitting model B, it is reasonable for Ni to share σ 2 and Δ R values with Al and silicon, even though Ni is a significantly heavier atom because when those variables are fit independently their error bars overlap with those of Ni [38] . In addition, using an isotropic expansion–contraction fitting model is reasonable to help reduce the number of independent fitting variables [38] . Others [11] , [16] have also restricted Δ R values of Ni and Al to be the same. The complications of shell-fitting analysis can be avoided in our sample runs by relying on the χ ( k ) × k 3 data. Although potentially better fits with the addition of silicon and/or Al can be achieved, the presence of Ni–Al LDH is indisputable because of the beat pattern and peak reduction at ~8.2 Å −1 present in all sample runs ( Figs 1 , 2 , 3 ). The rapid kinetics of metal adsorption and precipitation shown in real-time is a fundamental advance to our growing understanding of how fast these geochemical processes can occur at the mineral–water interface. Modelling of coprecipitation generally focused on the hydrolysis of the solvated cation (adsorptive) and not on hydrolysis of the cation dissolved from the sorbent; this model limits the adsorptive to the surface of the adsorbent and does not account for the formation of precipitates independent of the adsorbent surface but which utilize cations dissolved from it [15] . This latter process is critical in the formation of secondary minerals such as LDHs as formation of precipitates is highly related to mineral surface dissolution, that is, more soluble minerals form precipitates faster [25] . Even in a flow environment, where re-adsorption of dissolved products is limited compared with classical batch reactions [17] , we show that re-incorporation of dissolved Al cations into LDH occurs. We provide in situ , real-time, molecular-scale data showing that precipitation and adsorption can occur on the same short timescale of minutes. Conceptual models for metal sorption at the mineral–water interface should explicitly include both mechanisms. These results help us reconsider the role of the mineral at the mineral–water interface by showing that it can be very dynamic. This dynamic interaction is not limited to our specific experimental conditions [39] . In many cases, we cannot consider the mineral (adsorbent) a stable surface even over the short timescales in which we carry out laboratory experiments because the cycling of metals between solution and solid phases is very rapid. Flow cell setup A flow environment has the benefit of removing non-sorbed products from the reaction versus a batch reaction where products and reactants are still able to resorb to the surface [17] . The flow cell was custom cut from solid plastic and had a Kapton tape sealed reaction window with dimensions 5 mm high × 20 mm wide × 3 mm thick. That volume was packed with a homogeneous mixture of pyrophyllite clay and glass beads. The bulk density of the clay/glass bead mixture was 1.59 g cc −1 on average. It was placed ~45° in the X-ray path and solution containing Ni was pumped through it. The influent solution was pumped via a peristaltic pump at a rate of ~0.5 ml min −1 . The solution influent for Runs 1 and 2 was pH 7.5±0.1, 3 mM Ni buffered with 40 mM HEPES and 100 mM NaNO 3 . The solution influent for Runs 3, 4 and 5 was pH 7.5±0.1, 3 mM Ni buffered with 50 mM HEPES. The buffer maintains the pH during the LDH hydrolysis reaction occurring in the flow cell and the influent stock solution open to ambient air. The minimum amount of buffer necessary was used. Despite changes in ionic strength, Fig. 3 illustrates that all samples yield Ni–Al LDH phases over time. At the end of the reaction time, the flow was stopped and data were continuously collected on the non-flowing (NF) sample to measure any changes under stagnant conditions. Slightly different reaction conditions were used in part owing to limitations of the beamline (for example, beam fills, dumps and detector limitations). The results showed the formation of LDH phases regardless of the slight differences in experimental runs ( Fig. 3 ). For Run 1, the Ni solution was pumped through the cell continuously for 12.5 h. Fluorescence data were collected continuously and also obtained under NF conditions for 15 min at the end of the 12.5 h. For Run 2, the reaction was carried out for 5 h and 20 min and then stopped for ~8 h, after which NF data were collected for 40 min. For Run 3, Ni solution was pumped for 74 min and then flow was stopped. NF data were then immediately collected for 70 min. For Runs 4 and 5, the reactions ran for 4 h before the flow was stopped and NF data were acquired. Control experiments without pyrophyllite (that is, just glass beads in the flow cell) showed no increase in edge jump over time and an edge jump 3.6% in size compared with edge jumps at the end of experimental runs. This indicates little signal from aqueous Ni in the flow cell, little Ni sorption to the glass beads and no increase in Ni sorption to the glass beads over the reaction. Preparation of pyrophyllite mineral The <0.5 μm fraction of several different sources of naturally occurring pyrophyllite (Ward’s Science) was obtained by centrifugation in water at room temperature assuming a particle density of 2.65 g cc −1 and taking into account the initial and final settlement radii, r 1 and r 2, respectively. Conical centrifuge tubes (50 ml) were used in a swing-bucket centrifuge. X-ray diffraction confirmed the major mineral to be pyrophyllite in all samples with minor impurities of quartz. The clays were washed once with 0.5 M NaNO 3 and then three times with 18.2-megohm water and freeze dried. The homogenous clay/glass bead mixture inside the flow cell was 4 or 8% pyrophyllite mixed with glass beads. Run 1 had 4% pyrophyllite, whereas Runs 2, 3, 4 and 5 had 8% pyrophyllite. The glass beads were 250–300 μm in diameter, or ≥1,250–1,500 times larger than the pyrophyllite clay. In addition, glass beads low in trace metals, specifically iron, were obtained in order to minimize any interference of trace metal fluorescence from the beads into the passivated implanted planar silicon detector during the EXAFS experiments. Borosilicate glass beads low in trace metals obtained from Mo-Sci Specialty products, L.L.C. (product number GL0179B5/250–300) were used. Beamline setup All XAS experiments were carried out at the NSLS beamline X18B in Q-XAS mode [31] . The monochromator was detuned ~30% and oscillated at approximately 0.5 Hz. To minimize the effects of monochromator glitches, the monochromator was rotated in the χ -direction. This action markedly decreased glitch intensity and separated one large glitch into several smaller ones. The smaller glitches moved up to higher energy, to ~11.5 Å −1 , where they were excluded from the FT window. Current-to-voltage amplifiers were set to a filter time of 3 or 1 ms, with different standards used at each filter time to obtain the amplitude reduction factor ( Table 1 ). Ni K-edge fluorescence was measured with a passivated implanted planar silicon detector. QEXAFS data processing To process the Q-XAS data from X18B, multiple steps are necessary before background subtraction and normalization because data are continuously collected both up and down in energy. An encoder is used to measure the monochromator angle and Ni foil scans are used to convert the encoder angle to energy (eV) using the first derivative of the Ni foil (8,333 eV). The continuous up and down scans were cut at high and low energies to separate individual EXAFS scans. This procedure was carried out using custom software available at X18B. Subsequently, the software packages Athena and Artemis [40] were used for normalization, background subtraction, deglitching where appropriate and shell-fitting analysis. Owing to a glitch in the monochromator, it was necessary to remove in general 4–5 consecutive points in the EXAFS spectrum from the data collected at the end of sample runs and occasionally up to 8–9 consecutive points from data collected at the beginning of sample runs. Generally up to a 0.15-Å −1 gap in data points is allowed or 3 points on a 0.05 Å −1 grid for deglitching [38] . The amplifier filter set to 1 or 3 ms caused the glitch to spread out in energy and only those points affected were removed. Shell-fitting analysis of QEXAFS data For all spectra FT was carried out on χ ( k ) × k 3 data over a k -range of 3–11.3 with a k weighting of 3. Hanning window widths of 1 and 0.3 were used for the forward and back FT, respectively. FEFF6L (ref. 41 ) was used to calculate theoretical scattering paths of Ni–O, Ni–Ni, Ni–Al and Ni–Si based on the structure of lizardite [42] . In the lizardite structure, Ni and Al were substituted for magnesium. Amplitude reduction factors of 0.99 or 0.91 were determined from aqueous Ni and Ni hydroxide standards for the filter times of 1 or 3 ms, respectively, and applied to all fitting paths ( Table 1 ). The amplitude reduction factor of 0.85 (ref. 13 ) for Ni–Al LDH and α-Ni(OH) 2 was also used here. How to cite this article: Siebecker, M. et al. Real-time QEXAFS spectroscopy measures rapid precipitate formation at the mineral–water interface. Nat. Commun. 5:5003 doi: 10.1038/ncomms6003 (2014).